Adiponectin regulates psoriasiform skin inflammation by suppressing IL-17 production from γδ-T cells Accumulating epidemiologic evidence has revealed that metabolic syndrome is an independent risk factor for psoriasis development and is associated with more severe psoriasis. Adiponectin, primarily recognized as a metabolic mediator of insulin sensitivity, has been newly drawing attention as a mediator of immune responses. Here we demonstrate that adiponectin regulates skin inflammation, especially IL-17-related psoriasiform dermatitis. Mice with adiponectin deficiency show severe psoriasiform skin inflammation with enhanced infiltration of IL-17-producing dermal Vγ4+γδ-T cells. Adiponectin directly acts on murine dermal γδ-T cells to suppress IL-17 synthesis via AdipoR1. We furthermore demonstrate here that the adiponectin level of skin tissue as well as subcutaneous fat is decreased in psoriasis patients. IL-17 production from human CD4- or CD8-positive T cells is also suppressed by adiponectin. Our data provide a regulatory role of adiponectin in skin inflammation, which would imply a mechanism underlying the relationship between psoriasis and metabolic disorders. Psoriasis is a common chronic inflammatory skin disease, affecting ∼ 2–3% of the world’s population, which is characterized by epidermal hyperplasia, inflammatory cell infiltration and vascular changes [1] , [2] . In the development of psoriasis, keratinocytes and immune cells interact with each other through the production of cytokines. This cellular interplay, especially via the interleukin (IL)-23/Th17 cytokine network, finally leads to psoriatic plaque formation. IL-23, secreted by dendritic cells, differentiates naive T cells into Th17 cells, and these activated Th17 cells further secrete IL-17A, IL-17F and IL-22, which finally cause keratinocyte proliferation [3] , [4] , [5] . The importance of the IL-23/Th17 axis has been also exemplified by the therapeutic efficacy of human monoclonal antibodies targeting IL-12/23p40 (ustekinumab), IL-17 (ixekizumab and secukinumab) and its receptor (brodalumab) [6] , [7] , [8] . Psoriasis has been long considered to be a skin-tropic and not life-threatening disease; however, it is now increasingly recognized that psoriasis inflammation is not limited to the skin but goes far beyond the skin, accompanying systemic inflammation [9] , [10] . Immune cells and cytokines, when released into the systemic circulation, may alter the function of endothelial and haematopoietic cells, leading to the increase in the risk of insulin resistance and atherosclerosis. This inflammatory cascade is named ‘psoriatic march’, and psoriasis patients are now considered to be at higher risk of developing metabolic syndrome [11] . Systemic inflammation induced by obesity and metabolic syndrome, in turn, could exacerbate local skin inflammation via blood flow, which may consequently expand psoriasis inflammation [12] . The link between local and systemic inflammation is further supported by recent vast reports focusing on the high percentages of psoriasis patients who have cardiovascular and metabolic comorbidities [12] , [13] , [14] , [15] , [16] , [17] . Adipose tissue, although considered as an organ for energy storage in the past, is now accepted as an active endocrine and immune organ, which produces various bioactive molecules, named adipokines [18] , [19] . These adipokines, in cooperation with macrophages and T cells, cause adipose tissue inflammation and finally develop metabolic syndrome. Among these adipokines, adiponectin is a representative and main mediator of metabolism [20] , [21] . Interestingly, recent reports regarding adiponectin have been focusing on a new feature of adiponectin, an aspect as a regulator of immune responses [22] , [23] . A number of experimental studies suggest that adiponectin attenuates excessive inflammatory responses in a variety of tissues, especially in obesity-associated states [24] , [25] , [26] . Roles of adiponectin in the development of psoriasis, one of the obesity-linked diseases as mentioned above, have been also discussed in the vast past epidemiologic reports [27] , [28] , [29] . Serum adiponectin levels are decreased in psoriasis patients compared with healthy controls and its levels increase along with the improvement of dermatitis after successful treatments, including anti-tumour necrosis factor (TNF)-α agents, suggesting that adiponectin negatively regulates psoriasis progression [30] , [31] . Adiponectin in vitro suppresses TNF-α, IL-6 and IL-12p40 production from THP-1 cells, and IL-6 production from normal human keratinocytes [30] . These results have led us to further investigate whether adiponectin actually influences psoriasis inflammation in vivo . In the past few years, a mouse model of psoriasiform dermatitis induced by topical imiquimod application, has been frequently used to examine the inflammatory responses of the skin [32] , [33] . In this model, mice are treated topically with imiquimod cream for 6 consecutive days. After 6 days, rapid inflammation is noted in murine skin that resembles the clinical manifestation and histopathology of human psoriasis. In addition, this model mirrors the cytokine profile of human psoriasis, especially that of the IL-23/Th17-related pathway. Although this model indeed demonstrates a simple and acute skin inflammation and is not sufficient to replicate a chronic and complex human condition, alongside human studies, this model would be provided as one of the established ways to understand the immunological aspects of human disease [34] . The purpose of this study is to elucidate the possible roles of adiponectin in the development of psoriasis, using imiquimod- and IL-23-induced murine models of psoriasiform dermatitis along with human samples. We show here that lack of adiponectin exacerbates psoriasis-like skin inflammation with excessive infiltration of IL-17-producing Vγ4+ dermal γδ-T cells. Furthermore, adiponectin directly acts on dermal γδ-T cells to suppress IL-17 production. These results are in agreement with human data displaying the decreased level of adiponectin in subcutaneous fat and skin tissue of psoriasis patients. We also demonstrate regulatory roles of adiponectin on human CD4- and CD8-positive T cells. Although numerous reports have reported anti-inflammatory aspects of adiponectin on a variety of cell types, our data provides new evidence that adiponectin also has an anti-inflammatory effect on T cells and regulates skin inflammation. Adiponectin deficiency exacerbates psoriasiform dermatitis To examine the role of endogenous adiponectin during psoriasiform skin inflammation in vivo , we first applied imiquimod cream on mouse back skin, and investigated the clinical and histopathological features of wild-type and adiponectin-deficient mice. We also applied imiquimod cream on mouse ear skin and evaluated ear thickness. We confirmed that there are no differences in the phenotype or cytokine expressions between mice applied with Vaseline and a cream containing isostearic acid (25% w/w), a major component of the vehicle cream of the imiquimod ( Supplementary Fig. 1 ). Thus, we used Vaseline as a control cream of imiquimod in this study. Adiponectin-deficient mice exhibited worse clinical outcome with more severe scales and thicker skin at day 4–6 of imiquimod treatment as compared with wild-type mice ( Fig. 1a ). Clinical scores for disease severity were calculated daily using a scoring system based on the clinical Psoriasis Area and Severity Index. Significant differences in disease severity and ear thickness were observed between wild-type and adiponectin-deficient mice from day 4 to 6 ( Fig. 1b ). Consistent with clinical scores, histological analyses of skin samples at day 5 of imiquimod treatment on mouse back skin showed more severe epidermal hyperplasia and more intense inflammatory cell infiltration in adiponectin-deficient mice as compared with wild-type mice ( Fig. 1c ). Immunohistochemistry analyses revealed that infiltrating cells in the upper dermis were CD3 or major histocompatibility complex class II positive, and that cell counts for these positive cells were significantly increased in adiponectin-deficient mice compared with wild-type mice ( Fig. 1d ). 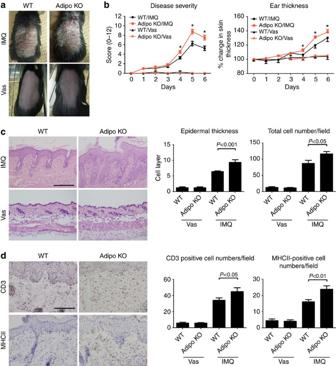Figure 1: Adiponectin deficiency promotes psoriasiform dermatitis. Shaved back skin and ears of wild-type (WT) and adiponectin-deficient (Adipo knockout (Adipo KO)) mice were topically treated with imiquimod (IMQ) or control Vaseline (Vas) for 6 consecutive days. (a) Phenotypical manifestation of WT and Adipo KO mouse back skin induced by IMQ or Ctrl cream application at day 5. (b) Disease severity (left panel) and ear thickness (right panel) during IMQ or Vas treatment. Clinical scores for disease severity were calculated daily using a scoring system based on the clinical Psoriasis Area and Severity Index. Data are presented as mean±s.e. (n=3–5 for each group). *P<0.05 versus WT mice with IMQ application. (c) Histological presentation of WT and Adipo KO mouse back skin induced by IMQ or Vas application at day 5 ( × 200). Scale bar, 50 μm. The number of epidermal cell layers and dermal inflammatory cells was counted per high-power field from 3 to 5 mice per group. Data are presented as mean±s.e. (n=3–5). (d) Immunohistochemical presentation of WT and Adipo KO mouse back skin induced by IMQ or Vas application at day 5 ( × 400). Scale bar, 25 μm. The number of CD3 or major histocompatibility complex (MHC) class II (MHCII)-positive cells was counted per high-power field from 3 to 5 mice per group. Data are presented as mean±s.e. (n=3–5), and analysed by Welch’st-test forb–d. Figure 1: Adiponectin deficiency promotes psoriasiform dermatitis. Shaved back skin and ears of wild-type (WT) and adiponectin-deficient (Adipo knockout (Adipo KO)) mice were topically treated with imiquimod (IMQ) or control Vaseline (Vas) for 6 consecutive days. ( a ) Phenotypical manifestation of WT and Adipo KO mouse back skin induced by IMQ or Ctrl cream application at day 5. ( b ) Disease severity (left panel) and ear thickness (right panel) during IMQ or Vas treatment. Clinical scores for disease severity were calculated daily using a scoring system based on the clinical Psoriasis Area and Severity Index. Data are presented as mean±s.e. ( n =3–5 for each group). * P <0.05 versus WT mice with IMQ application. ( c ) Histological presentation of WT and Adipo KO mouse back skin induced by IMQ or Vas application at day 5 ( × 200). Scale bar, 50 μm. The number of epidermal cell layers and dermal inflammatory cells was counted per high-power field from 3 to 5 mice per group. Data are presented as mean±s.e. ( n =3–5). ( d ) Immunohistochemical presentation of WT and Adipo KO mouse back skin induced by IMQ or Vas application at day 5 ( × 400). Scale bar, 25 μm. The number of CD3 or major histocompatibility complex (MHC) class II (MHCII)-positive cells was counted per high-power field from 3 to 5 mice per group. Data are presented as mean±s.e. ( n =3–5), and analysed by Welch’s t -test for b – d . Full size image Adiponectin deficiency promotes IL-17A gene expression We next examined the messenger RNA (mRNA) expression levels of psoriasis-related cytokines in the imiquimod-induced psoriasiform skin lesions of wild-type and adiponectin-deficient mice. Skin samples were taken from mouse back skin, before treatment, and 24 or 48 h after imiquimod application. Messenger RNA levels for TNF-α, IFN-γ, IL-6, IL-12p40, IL-23p19, IL-17A, IL-17F and IL-22 were determined by quantitative real-time PCR. Imiquimod-treated skin demonstrated increased mRNA levels of genes mentioned above, and adiponectin deficiency further augmented mRNA levels of TNF-α, IL-6, IL-12p40 and IL-23p19, which would reflect the anti-inflammatory roles of adiponectin on macrophages and dendritic cells. In addition, mRNA levels of IL-17A, IL-17F and IL-22 were also markedly upregulated in adiponectin-deficient mice at 48 h after imiquimod application, as compared with wild-type mice ( Fig. 2a ). In the experiment of intradermal IL-23 injections to mouse ear skin, another widely used model of psoriasiform skin inflammation, IL-17A/IL-17F/IL-22 expression was upregulated after IL-23 injection [33] , [35] , and adiponectin deficiency further increased their expression level ( Fig. 2b ). Interestingly, IL-17A expression was much greater with IL-23 injection than imiquimod treatment, whereas IL-17F and IL-22 were far less responsive to IL-23 injection than to imiquimod treatment in adiponectin-deficient mice, suggesting that the major effect of adiponectin is on IL-17A. Thus, we sought to focus on the effect of adiponectin especially on IL-17A. Notably, there was great increase in both IL-6 and IL-17A expression in adiponectin-deficient mice at 48 h after imiquimod application ( Fig. 2a ). In detail, IL-6 was sufficiently produced after 24 h of imiquimod application, whereas IL-17A was gradually produced until 48 h in adiponectin-deficient mice, suggesting the possibility that IL-6 overproduction in adiponectin-deficient mice might predominate further increase in IL-17A production at 48 h. To address this concern, we conducted an intraperitoneal injection of IL-6 antibody in both adiponectin-deficient and wild-type mice, and then compared IL-17A expression level 48 h after imiquimod application. As shown in Fig. 2c , IL-6 antibody injection suppressed, but not significantly, about half of IL-17A production in wild-type mice. In adiponectin-deficient mice, suppression level of IL-17A by IL-6 antibody was more remarkable as compared with that in wild-type mice. This result would imply that the IL-17A production might be regulated partially by IL-6 in the imiquimod-induced skin inflammation and that the enhanced IL-6 production by adiponectin deficiency might induce subsequent IL-17A production and exacerbation of dermatitis. 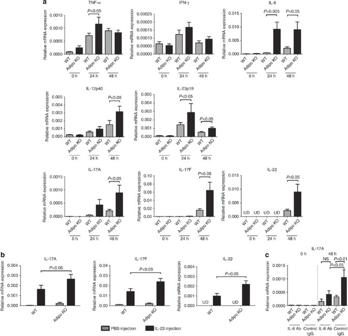Figure 2: Adiponectin deficiency promotes gene expression of cytokines implicated in the psoriasiform skin inflammation. Wild-type (WT) and Adiponectin knockout (Adipo KO) mice were (a) applied with imiquimod (IMQ) or (b) injected with IL-23 intradermally, and skin samples were taken (a) before treatment, and 24 or 48 h after IMQ application or (b) after second IL-23 injection. Messenger RNA levels of the indicated cytokines were determined by quantitative PCR. Data are obtained from duplicate samples from 5 to 8 mice in each group. Values are presented as mean±s.e. (n=10–16). UD, undetected. (c) WT and Adipo KO mice were injected with IL-6 antibody intraperitoneally, and IL-17A mRNA level of skin samples was determined before treatment and 48 h after IMQ application. Data are obtained from duplicate samples from 2 to 4 mice in each group. Values are presented as mean±s.e. (n=4: 0 h,n=8: 48 h). Data are analysed by Welch’st-test fora,band by one-way analysis of variance with Dunnett’s multiple comparison test forc. NS, not significant. Figure 2: Adiponectin deficiency promotes gene expression of cytokines implicated in the psoriasiform skin inflammation. Wild-type (WT) and Adiponectin knockout (Adipo KO) mice were ( a ) applied with imiquimod (IMQ) or ( b ) injected with IL-23 intradermally, and skin samples were taken ( a ) before treatment, and 24 or 48 h after IMQ application or ( b ) after second IL-23 injection. Messenger RNA levels of the indicated cytokines were determined by quantitative PCR. Data are obtained from duplicate samples from 5 to 8 mice in each group. Values are presented as mean±s.e. ( n =10–16). UD, undetected. ( c ) WT and Adipo KO mice were injected with IL-6 antibody intraperitoneally, and IL-17A mRNA level of skin samples was determined before treatment and 48 h after IMQ application. Data are obtained from duplicate samples from 2 to 4 mice in each group. Values are presented as mean±s.e. ( n =4: 0 h, n =8: 48 h). Data are analysed by Welch’s t -test for a , b and by one-way analysis of variance with Dunnett’s multiple comparison test for c . NS, not significant. Full size image Adiponectin regulates IL-17A-producing dermal γδ-T cells To clarify whether adiponectin deficiency is actually involved in the local skin inflammation, we next performed intracellular flow cytometric analyses of the skin after imiquimod application. Single-cell suspensions from the dermis separated from the epidermis of wild-type and adiponectin-deficient mice after 5 days of imiquimod treatment were stimulated with phorbol 12-myristate 13-acetate (PMA) and ionomycin, and then were analysed for IL-17A as well as CD3 and γδTCR expression. Adiponectin deficiency promoted the recruitment of CD3-positive cells to the dermis of imiquimod-induced skin as compared with wild-type mice ( Fig. 3a,b ). The proportion of γδ-T cells among these infiltrating CD3-positive cells was similar between wild-type and adiponectin-deficient mice ( Fig. 3c,d ). In addition, as well as increased infiltrating CD3-positive cells, expression levels of IL-17A on a per-cell basis among CD3-positive cells were also significantly increased in adiponectin-deficient mice ( Fig. 3e,g ). Next, we gated on IL-17-positive cells and determined the cellular source of IL-17. In agreement with previous reports [33] , [36] , the majority of IL-17 was produced by γδ-T cells upon stimulation ( Fig. 3f,h ). These results suggest that adiponectin deficiency promotes the recruitment of inflammatory cells and local IL-17 production from γδ-T cells in the imiquimod-induced skin inflammation. 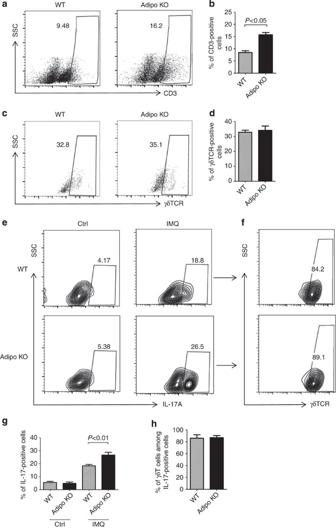Figure 3: Adiponectin negatively regulates the recruitment of inflammatory cells and the IL-17 production from γδ-T cells in the skin. Wild-type (WT) and Adiponectin knockout (Adipo KO) mice were treated as described. At day 5, dermal cell suspensions of mouse back skin were stimulated with PMA and ionomycin, and were stained with antibodies specific for IL-17A as well as CD3 and TCRγδ cell surface markers, followed by flow cytometric analysis. Gating stragedy is shown inSupplementary Fig. 3. (a,c,e,f) Flow plots show the CD3-positive (a), TCRγδ-positive (c,f), IL-17A-positive (e) population of the dermal cells from WT and Adipo KO mice. Flow plots were gated on CD3-positive cells (c,e). (b,d,g,h) Graph shows the percentage of CD3-positive (b), TCRγδ-positive (d,h) and IL-17-positive (g) cells. The percentage of IL-17-positive cells among CD3 cells of each group is shown inSupplementary Table 1. Values are presented as mean±s.e. (n=6). Data are representative of three independent experiments, where each group contains 1 to 2 mice. Data are analysed by Welch’st-test fora,b,g,h. IMQ, imiquimod. Figure 3: Adiponectin negatively regulates the recruitment of inflammatory cells and the IL-17 production from γδ-T cells in the skin. Wild-type (WT) and Adiponectin knockout (Adipo KO) mice were treated as described. At day 5, dermal cell suspensions of mouse back skin were stimulated with PMA and ionomycin, and were stained with antibodies specific for IL-17A as well as CD3 and TCRγδ cell surface markers, followed by flow cytometric analysis. Gating stragedy is shown in Supplementary Fig. 3 . ( a , c , e , f ) Flow plots show the CD3-positive ( a ), TCRγδ-positive ( c , f ), IL-17A-positive ( e ) population of the dermal cells from WT and Adipo KO mice. Flow plots were gated on CD3-positive cells ( c , e ). ( b , d , g , h ) Graph shows the percentage of CD3-positive ( b ), TCRγδ-positive ( d , h ) and IL-17-positive ( g ) cells. The percentage of IL-17-positive cells among CD3 cells of each group is shown in Supplementary Table 1 . Values are presented as mean±s.e. ( n =6). Data are representative of three independent experiments, where each group contains 1 to 2 mice. Data are analysed by Welch’s t -test for a , b , g , h . IMQ, imiquimod. Full size image Vγ4-positive dermal γδ-T cells are the major IL-17 producers To determine which type of γδ-T cells are involved in the dermal skin inflammation, we examined the Vγ4 and Vγ5 expression pattern of skin γδ-T cells during the imiquimod treatment. We first determined the Vγ4 and Vγ5 expression of epidermal resident γδ-T cells and dermal migratory γδ-T cells by reverse transcription–PCR. As shown in Fig. 4a , dermal γδ-T cells expressed Vγ4, whereas epidermal γδ-T cells express Vγ5, but not Vγ4. Notably, imiquimod application induced two subsets of skin γδ-T cells, composed of TCRγδ intermidiate IL-17+(I) and TCRγδ high IL-17-(II) T cells in both wild-type and adiponectin-deficient mice ( Fig. 4b ). Consistent with the past reports [33] , [37] , [38] , these populations expressed (I) Vγ4 and (II) Vγ5, respectively ( Fig. 4c ), suggesting that Vγ4-positive dermal migratory γδ-T cells dominate the dermal skin inflammation and IL-17 production. In accordance with this result, when gated on IL-17-positive cell subsets, the majority of IL-17-positive cells expressed Vγ4, but not Vγ5, in both wild-type and adiponectin-deficient mice ( Fig. 4d ). 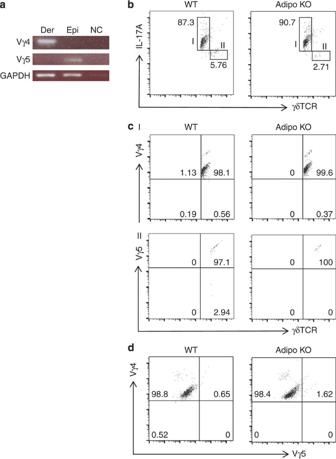Figure 4: Vγ4 T cells predominantly induce the skin inflammation and are the major IL-17 producers. Wild-type (WT) and Adiponectin knockout (Adipo KO) mice were treated as described. At day 5, whole-skin cell suspensions of mouse back skin were stimulated with PMA and ionomycin, and were stained with antibodies specific for IL-17A as well as CD3, TCRγδ, Vγ4 and Vγ5 cell surface markers, followed by flow cytometric analysis. (a) Dermal γδ-T cells after IMQ application and epidermal γδ-T cells before IMQ application were sorted, and mRNAs were extracted to perform reverse transcription–PCR. (b) Plots show two populations of γδ-T cells, composed of TCRγδintermediateIL-17-positive (I) and TCRγδhighIL-17-negative (II) cells. (c) Cells of (I) and (II) populations were characterized for TCRγδ and Vγ4 or Vγ5 expression. (d) IL-17-positive cells gated on CD3-positive cells were characterized for Vγ4 and Vγ5 expression. Data are representative of two independent experiments, where each group contains two mice. Figure 4: Vγ4 T cells predominantly induce the skin inflammation and are the major IL-17 producers. Wild-type (WT) and Adiponectin knockout (Adipo KO) mice were treated as described. At day 5, whole-skin cell suspensions of mouse back skin were stimulated with PMA and ionomycin, and were stained with antibodies specific for IL-17A as well as CD3, TCRγδ, Vγ4 and Vγ5 cell surface markers, followed by flow cytometric analysis. ( a ) Dermal γδ-T cells after IMQ application and epidermal γδ-T cells before IMQ application were sorted, and mRNAs were extracted to perform reverse transcription–PCR. ( b ) Plots show two populations of γδ-T cells, composed of TCRγδ intermediate IL-17-positive (I) and TCRγδ high IL-17-negative (II) cells. ( c ) Cells of (I) and (II) populations were characterized for TCRγδ and Vγ4 or Vγ5 expression. ( d ) IL-17-positive cells gated on CD3-positive cells were characterized for Vγ4 and Vγ5 expression. Data are representative of two independent experiments, where each group contains two mice. Full size image IL-17 regulation in γδ-T cells is mediated through AdipoR1 We next focused on the in vitro effects of adiponectin on dermal γδ-T cells. First of all, we examined the expression of adiponectin receptors, AdipoR1 and AdipoR2. It is known that AdipoR1 is expressed widely in various tissues, while AdipoR2 is predominantly expressed in the liver [39] . As shown in Fig. 5a , western blot analysis demonstrated that only AdipoR1 protein was detected, while AdipoR2 protein expression was below the detection limit. Next, we investigated whether adiponectin had a direct effect on the production of IL-17 by γδ-T cells. Sorted dermal γδ-T cells were pretreated with indicated concentrations of adiponectin for 1 h, followed by treatment with IL-1β (10 ng ml −1 ) and IL-23 (5 ng ml −1 ) for another 24 h, and IL-17 protein levels in the supernatant were quantified. We confirmed that adiponectin itself was not harmful by determining that IL-2 production of dermal γδ-T cells is not influenced by adiponectin concentration up to 50 μg ml −1 ( Supplementary Fig. 2a ). Since earlier studies have revealed that γδ-T cells express IL-23R and produce IL-17 in response to IL-1β and IL-23 (ref. 40 ), without T-cell receptor engagement, we incubated γδ-T cells without activation by anti-CD3e monoclonal antibody in this experiment. As shown in Fig. 5b , adiponectin directly suppressed IL-17 production from dermal γδ-T cells in a dose-dependent manner up to 25 μg ml −1 . Consistent with the result of the supernatant protein levels, pretreatment with adiponectin (10 μg ml −1 ) suppressed IL-17A mRNA expression of dermal γδ-T cells ( Fig. 5c ). Furthermore, to determine which adiponectin receptor, AdipoR1 or AdipoR2, is involved in the regulation of IL-17 synthesis, dermal γδ-T cells were transfected with short interfering RNA (siRNA) against AdipoR1 and AdipoR2, and thereafter, were assessed for IL-17A mRNA expression. Quantitative real-time PCR detected both AdipoR1 and AdipoR2 mRNA in dermal γδ-T cells, although AdipoR2 protein expression was below the detection limit by western blot analysis. This result is consistent with the past reports demonstrating discrepancy between mRNA and protein levels of AdipoR2 in leukocytes [41] , [42] . Control experiments have revealed that AdipoR1 and AdipoR2 mRNA levels are reduced by >65% as evaluated by real-time reverse transcription–PCR analysis ( Fig. 5d ). We found that specific knockdown of AdipoR1, but not of AdipoR2, attenuated suppression of adiponectin-induced IL-17A gene expression in dermal γδ-T cells ( Fig. 5e ), indicating that adiponectin suppresses IL-17 synthesis through AdipoR1 in dermal γδ-T cells. Again, IL-2 expression of γδ-T cells stimulated with IL-1β and IL-23 was not influenced by treatment with adiponectin ( Supplementary Fig. 2b ). 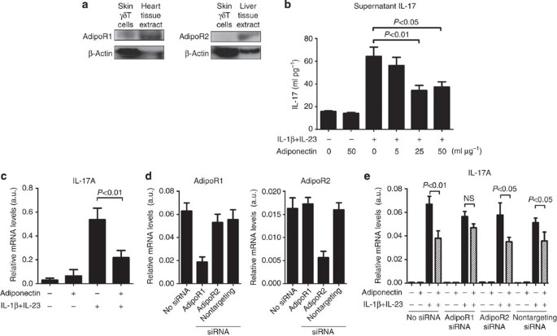Figure 5: Adiponectin negatively regulates IL-17 production from dermal γδ-T cells through AdipoR1. (a) Sorted dermal γδ-T cells were analysed for the expression of adiponectin receptors, AdipoR1 and AdipoR2. Mouse heart and liver extract were used as a positive control, respectively. (b,c) Dermal γδ-T cells were pretreated with indicated concentrations of adiponectin for 1 h, followed by treatment with IL-1β (10 ng ml−1) and IL-23 (5 ng ml−1) (b) for another 24 h, and the supernatant IL-17 levels were determined using the IL-17 ELISA kit (n=5: cells without IL-1β and IL-23 stimulation,n=6: cells with IL-1β and IL-23 stimulation), and (c) for another 6 h, and the gene expression levels of IL-17A was determined by quantitative (qPCR) (n=4: cells without IL-1β and IL-23 stimulation,n=5: cells with IL-1β and IL-23 stimulation). Data are mean±s.e. and are representative of two independent experiments. (d,e) Dermal γδ-T cells were transfected with AdipoR1 or AdipoR2 siRNA or nontargeting control siRNA. After 72 h, γδ-T cells were pretreated with adiponectin (10 μg ml−1) for 1 h, followed by treatment with IL-1β (10 ng ml−1) and IL-23 (5 ng ml−1) for another 6 h. Messenger RNA expression of (d) AdipoR1 and AdipoR2 (n=8) and (e) IL-17A (n=4: cells without IL-1β and IL-23 stimulation,n=6: cells with IL-1β and IL-23 stimulation) in transfected cells were examined by qPCR. Data are mean±s.e. and are representative of three independent experiments. Data are analysed by Welch’st-test forb,c,e. NS, not significant. Figure 5: Adiponectin negatively regulates IL-17 production from dermal γδ-T cells through AdipoR1. ( a ) Sorted dermal γδ-T cells were analysed for the expression of adiponectin receptors, AdipoR1 and AdipoR2. Mouse heart and liver extract were used as a positive control, respectively. ( b , c ) Dermal γδ-T cells were pretreated with indicated concentrations of adiponectin for 1 h, followed by treatment with IL-1β (10 ng ml −1 ) and IL-23 (5 ng ml −1 ) ( b ) for another 24 h, and the supernatant IL-17 levels were determined using the IL-17 ELISA kit ( n =5: cells without IL-1β and IL-23 stimulation, n =6: cells with IL-1β and IL-23 stimulation), and ( c ) for another 6 h, and the gene expression levels of IL-17A was determined by quantitative (qPCR) ( n =4: cells without IL-1β and IL-23 stimulation, n =5: cells with IL-1β and IL-23 stimulation). Data are mean±s.e. and are representative of two independent experiments. ( d , e ) Dermal γδ-T cells were transfected with AdipoR1 or AdipoR2 siRNA or nontargeting control siRNA. After 72 h, γδ-T cells were pretreated with adiponectin (10 μg ml −1 ) for 1 h, followed by treatment with IL-1β (10 ng ml −1 ) and IL-23 (5 ng ml −1 ) for another 6 h. Messenger RNA expression of ( d ) AdipoR1 and AdipoR2 ( n =8) and ( e ) IL-17A ( n =4: cells without IL-1β and IL-23 stimulation, n =6: cells with IL-1β and IL-23 stimulation) in transfected cells were examined by qPCR. Data are mean±s.e. and are representative of three independent experiments. Data are analysed by Welch’s t -test for b , c , e . NS, not significant. Full size image Exogenous adiponectin rescues exacerbated dermatitis To determine whether the exacerbation of dermatitis in adiponectin-deficient mice is particularly adiponectin dependent or not, wild-type and adiponectin-deficient mice were given daily intraperitoneal injection of adiponectin (50 μg per day per mouse) [15] from 1 day before imiquimod treatment, and the dermatitis progression and IL-17 expression were examined. Exogenous adiponectin improved imiquimod-induced dermatitis clinically and pathologically ( Fig. 6a ). Disease severity and ear thickness during imiquimod treatment are shown in Fig. 6b,c . Consistent with the improvement of the phenotype, exogenous adiponectin significantly suppressed elevated IL-17 production of adiponectin-deficient mice ( Fig. 6d ). On the other hand, additional adiponectin did not either suppress IL-17 production or improve dermatitis of wild-type mice ( Fig. 6a–d ). These results would suggest that the effect of adiponectin might be elicited below a certain concentration of adiponectin and that exogenous adiponectin supplementation could be effective only under the condition when adiponectin is insufficient, implying the existence of a plateau concentration that would exert biological effects in vivo . 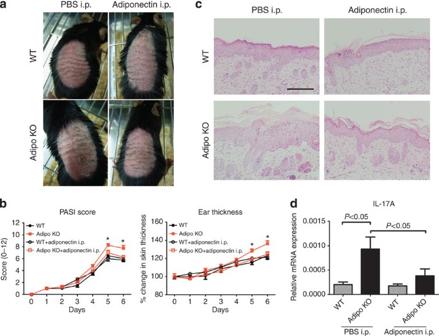Figure 6: Exogenous adiponectin improves the psoriasiform dermatitis in Adipo knockout (KO) mice. Wild-type (WT) and Adiponectin knockout (Adipo KO) mice were given daily intraperitoneal (i.p.) injection of recombinant adiponectin (50 μg per day) from day 1 before imiquimod (IMQ) treatment. (a) Phenotypical manifestation of WT and Adipo KO mouse back skin induced by IMQ at day 5 with or without exogenous adiponectin administration. (b) Disease severity (left panel) and ear thickness (right panel) during IMQ treatment. Clinical scores for disease severity were calculated as described in the Methods. Data are presented as mean±s.e. (n=4 for each group). *P<0.05 versus Adipo KO mice without adiponectin administration. Data are analysed by Welch’st-test. (c) Histological presentation of WT and Adipo KO mouse back skin induced by IMQ at day 5 with or without exogenous adiponectin administration. Scale bar, 50 μm. (d) IL-17 mRNA expression of WT and Adipo KO mouse back skin induced by IMQ at day 2 with or without exogenous adiponectin administration. Data are analysed by one-way analysis of variance with Dunnett’s multiple comparison test. Figure 6: Exogenous adiponectin improves the psoriasiform dermatitis in Adipo knockout (KO) mice. Wild-type (WT) and Adiponectin knockout (Adipo KO) mice were given daily intraperitoneal (i.p.) injection of recombinant adiponectin (50 μg per day) from day 1 before imiquimod (IMQ) treatment. ( a ) Phenotypical manifestation of WT and Adipo KO mouse back skin induced by IMQ at day 5 with or without exogenous adiponectin administration. ( b ) Disease severity (left panel) and ear thickness (right panel) during IMQ treatment. Clinical scores for disease severity were calculated as described in the Methods. Data are presented as mean±s.e. ( n =4 for each group). * P <0.05 versus Adipo KO mice without adiponectin administration. Data are analysed by Welch’s t -test. ( c ) Histological presentation of WT and Adipo KO mouse back skin induced by IMQ at day 5 with or without exogenous adiponectin administration. Scale bar, 50 μm. ( d ) IL-17 mRNA expression of WT and Adipo KO mouse back skin induced by IMQ at day 2 with or without exogenous adiponectin administration. Data are analysed by one-way analysis of variance with Dunnett’s multiple comparison test. Full size image Neutralization of IL-17 ameliorates exacerbated dermatitis Finally, to assess clinical effectiveness, wild-type and adiponectin-deficient mice were intraperitoneally injected with high (80 μg) or low (10 μg) doses of anti-IL-17 antibody, and then were applied imiquimod cream for 6 consecutive days. As shown in Fig. 7a , adiponectin-deficient mice with low doses of anti-IL-17 antibody injection revealed no visible phenotypic changes. In contrast, wild-type mice demonstrated phenotypical improvement with both low and high doses injection of anti-IL-17 antibody. Disease severity and ear thickness (lower panel) during imiquimod treatment are shown in Fig. 7b . Histological presentation was consistent with these phenotypes. Specifically, epidermal hyperplasia and inflammatory cell infiltration were improved in wild-type mice with both low- and high-dose injections, but in adiponectin-deficient mice with only high-dose injection ( Fig. 7c ). 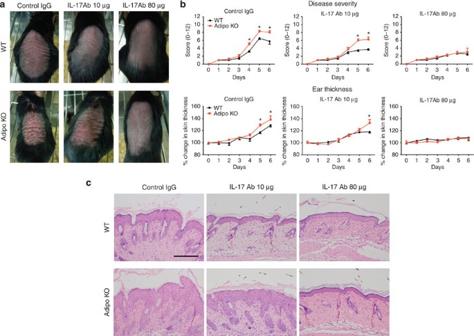Figure 7: Adipo knockout (KO) mice need a further dose of anti-IL-17 antibody to prevent the psoriasiform dermatitis. Wild-type (WT) and Adipo KO mice were intraperitoneally injected with control IgG, or 10 and 80 μg of anti-IL-17 antibody (IL-17 Ab) at 1 day before (day −1) and 2 days after (day 2) imiquimod (IMQ) treatment. (a) Phenotypical manifestation of WT and Adipo KO mouse back skin induced by IMQ at day 5. (b) Disease severity (upper panel) and ear thickness (lower panel) during IMQ treatment. Clinical scores for disease severity were calculated as described in the Methods. Data are presented as mean±s.e. (n=4 for each group). *P<0.05 versus WT mice with IMQ application. Data are analysed by Welch’st-test. (c) Histological presentation of WT and Adipo KO mouse back skin induced by IMQ at day 5 with the indicated dose of IL-17 antibody injection. Scale bar, 50 μm. Figure 7: Adipo knockout (KO) mice need a further dose of anti-IL-17 antibody to prevent the psoriasiform dermatitis. Wild-type (WT) and Adipo KO mice were intraperitoneally injected with control IgG, or 10 and 80 μg of anti-IL-17 antibody (IL-17 Ab) at 1 day before (day −1) and 2 days after (day 2) imiquimod (IMQ) treatment. ( a ) Phenotypical manifestation of WT and Adipo KO mouse back skin induced by IMQ at day 5. ( b ) Disease severity (upper panel) and ear thickness (lower panel) during IMQ treatment. Clinical scores for disease severity were calculated as described in the Methods. Data are presented as mean±s.e. ( n =4 for each group). * P <0.05 versus WT mice with IMQ application. Data are analysed by Welch’s t -test. ( c ) Histological presentation of WT and Adipo KO mouse back skin induced by IMQ at day 5 with the indicated dose of IL-17 antibody injection. Scale bar, 50 μm. Full size image Effects of adiponectin on human T cells To determine whether obtained murine data are in accordance with human condition, we collected human skin and subcutaneous samples of psoriasis patients as well as controls, and compared its adiponectin level. Notably, adiponectin level of subcutaneous fat was remarkably decreased in psoriasis patients as compared with healthy controls ( Fig. 8a , left panel). Furthermore, adiponectin levels of skin tissue, which locate directly above subcutaneous adipose tissue, were also significantly decreased in psoriasis patients ( Fig. 8a , right panel). Adiponectin level of skin tissue significantly correlated with that of subcutaneous fat tissue in individual patients ( Fig. 8b ). Since conventional CD4- or CD8-positive T cells dominantly infiltrate the dermis of psoriasis patients and contribute to the formation of psoriasis plaque, we sought to examine whether adiponectin actually suppresses IL-17 production by human CD4- or CD8-positive T cells. Human CD4- and CD8-positive T cells expressed adiponectin receptor, AdipoR1, but not AdipoR2, at the protein level ( Fig. 8c ). Peripheral blood mononuclear cells (PBMCs) were activated with IL-23 (0 and 25 ng ml −1 ), plate-bound anti-CD3 and soluble anti-CD28 with pretreatment of indicated concentrations of adiponectin. IL-17 production by PBMC was inhibited by adiponectin, in a dose-dependent manner up to 25 μg ml −1 ( Fig. 8d ). We also determined the percentage of IL-17-positive cells among CD4- or CD8-positive T cells, activated as mentioned above with or without adiponectin (25 μg ml −1 ) pretreatment. Flow cytometric analyses revealed the inhibitory effects of adiponectin on human CD4- and CD8-positive T cells ( Fig. 8e,f ). 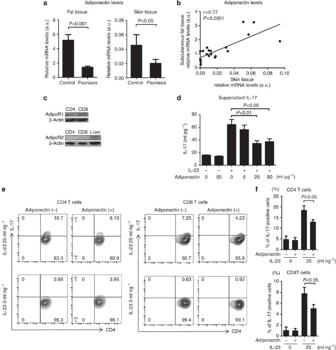Figure 8: Adiponectin suppresses IL-17 production from human CD4- and CD8-positive T cells. (a) Messenger RNAs of subcutaneous fat (left panel) and skin (middle panel) tissue from psoriasis patients (n=26) and healthy controls (n=12) were extracted and examined for adiponectin level by quantitative (q)PCR. Data are mean±s.e. and analysed by Welch’st-test. (b) Correlation of adiponectin level in psoriasis patients between subcutaneous fat and skin tissue is shown in the right panel. (c) Human CD4 and CD8-positive T cells were sorted and were analysed for the expression of adiponectin receptors, AdipoR1 and AdipoR2. (d) PBMCs were obtained from human whole blood, and were pretreated with indicated concentrations of adiponectin for 1 h, followed by treatment with plate-bound anti-CD3(5 μg ml−1), soluble anri-CD28 (1 μg ml−1) and IL-23 (0 and 25 ng ml−1) for another 7 days. The supernatant IL-17 levels were determined using the IL-17 ELISA kit. Data are mean±s.e. (n=4) and are representative of two independent experiments. Data are analysed by one-way analysis of variance with Dunnett’s multiple comparison test. (e) Human PBMCs were treated as mentioned above for 5 days, stimulated with PMA and ionomycin and were stained with antibodies specific for IL-17A as well as CD4 and CD8 cell surface markers, followed by flow cytometric analysis. Data are representative of three independent experiments. (f) Graph shows the percentage of IL-17-positive cells among CD4- or CD8-positive T cells (n=3: IL-23 0 ng ml−1,n=6: IL-23 25 ng ml−1). Data are analysed by Welch’st-test. Figure 8: Adiponectin suppresses IL-17 production from human CD4- and CD8-positive T cells. ( a ) Messenger RNAs of subcutaneous fat (left panel) and skin (middle panel) tissue from psoriasis patients ( n =26) and healthy controls ( n =12) were extracted and examined for adiponectin level by quantitative (q)PCR. Data are mean±s.e. and analysed by Welch’s t -test. ( b ) Correlation of adiponectin level in psoriasis patients between subcutaneous fat and skin tissue is shown in the right panel. ( c ) Human CD4 and CD8-positive T cells were sorted and were analysed for the expression of adiponectin receptors, AdipoR1 and AdipoR2. ( d ) PBMCs were obtained from human whole blood, and were pretreated with indicated concentrations of adiponectin for 1 h, followed by treatment with plate-bound anti-CD3(5 μg ml −1 ), soluble anri-CD28 (1 μg ml −1 ) and IL-23 (0 and 25 ng ml −1 ) for another 7 days. The supernatant IL-17 levels were determined using the IL-17 ELISA kit. Data are mean±s.e. ( n =4) and are representative of two independent experiments. Data are analysed by one-way analysis of variance with Dunnett’s multiple comparison test. ( e ) Human PBMCs were treated as mentioned above for 5 days, stimulated with PMA and ionomycin and were stained with antibodies specific for IL-17A as well as CD4 and CD8 cell surface markers, followed by flow cytometric analysis. Data are representative of three independent experiments. ( f ) Graph shows the percentage of IL-17-positive cells among CD4- or CD8-positive T cells ( n =3: IL-23 0 ng ml −1 , n =6: IL-23 25 ng ml −1 ). Data are analysed by Welch’s t -test. Full size image A number of epidemiologic studies have been focusing on the close relationship between psoriasis and metabolic disorders in terms of adipokines, including adiponectin. However, specific roles of adiponectin in the regulation of skin immune responses remain to be unknown. Using a mouse model of psoriasiform dermatitis, alongside human samples, we set out to determine whether and how adiponectin is involved in the immunological development of psoriasiform skin inflammation in this study. First of all, to confirm that there is not a baseline difference in cutaneous immune responses or epithelia between wild-type and adiponectin-deficient mice, we have conduced contact hypersensitivity experiments on these mice using 2,4-dinitrofluorobenzene or fluorescein isothiocyanate. As shown in Supplementary Fig. 4 , no significant difference was observed in mouse ear thickness between these mice in both 2,4-dinitrofluorobenzene- and fluorescein isothiocyanate-applied conditions. We observed that adiponectin deficiency resulted in severe psoriasiform inflammation. Since it is widely known that inhibition of adiponectin upregulates TNF-α production from macrophages or adipocytes [25] , [43] , we expected that the increased skin inflammation in adiponectin-deficient mice was mainly due to the overexpression of TNF-α. Although TNF-α expression was indeed elevated in the inflamed skin of adiponectin-deficient mice, even more striking was the upregulated expression of Th17-related cytokines, IL-17A/IL-17F/IL-22. The regulation of IL-17 by adiponectin was strengthened by the flow cytometric analysis, in which adiponectin deficiency caused increased amount of IL-17 expression by CD3-positive cells on a per-cell basis, along with enhanced recruitment of CD3-positive cells to the skin. In addition, adiponectin exerts a direct suppressive effect on the production of IL-17. Since IL-17 plays central roles in the pathogenesis and maintenance of psoriasis, it could be speculated that adiponectin deficiency would drive skin inflammation, especially IL-17-related psoriasiform inflammation. In the analyses of human samples, psoriasis patients displayed decreased adiponectin levels at both subcutaneous fat and skin site, suggesting that psoriasis patients possess a condition predisposed to produce IL-17 and develop subsequent dermatitis. Although anti-inflammatory properties of adiponectin have been well-investigated and discussed, most reports have been focusing on the relation between adiponectin and TNF-α or IL-6. Adiponectin suppresses TNF-α or IL-6 production and TNF-α-induced biological effects of certain cells, such as adipocytes, macrophages, endothelial cells and hepatocytes [23] , [43] , [44] , [45] . These anti-inflammatory and suppressive effects of adiponectin against TNF-α and IL-6 are involved in the pathogenesis of life-related diseases, such as atherosclerosis, insulin resistance or alcoholic/non-alcoholic liver disease, in which these cytokines act as main players in the disease development [46] , [47] , [48] . However, there still exist few reports investigating the function of adiponectin in the regulation of IL-17. Two reports with different disease models have shown the enhanced IL-17 production and disease exacerbation in adiponectin-deficient mice. In the mouse model of multiple sclerosis, which is another representative Th17-related disease, adiponectin-deficient mice developed worse experimental autoimmune encephalomyelitis with higher IL-17 expression of spinal cord tissues [49] . Another report can be obtained from an ozone-induced pulmonary inflammation model, one of the mouse models for asthma, in which adiponectin-deficient mice showed increased ozone-induced inflammation and IL-17A expression in the lung [50] . In the present study, adiponectin-deficient mice developed worse psoriasis inflammation with increased IL-17 expression of the skin, strengthening the hypothesis that adiponectin possesses anti-inflammatory properties in the regulation of IL-17. Another point to be focused on is a time course of IL-6 and IL-17A expression. In the imiquimod-induced skin inflammation, IL-6 expression was first enhanced and thereafter IL-17A expression was upregulated. In addition, IL-6 depletion by IL-6 antibody attenuated about half of IL-17A expression, suggesting that IL-6 might regulate the subsequent IL-17A expression. The function of IL-6 in the differentiation of IL-17A-producing γδ-T cells, which are main producers of IL-17A in the imiquimod-induced dermatitis, is still controversial [51] , [52] . It has been reported that IL-6-deficient mice showed a twofold decrease in the percentage of IL-17A+ cells [51] , suggesting a partial contribution of IL-6 in the IL-17A production by γδ-T cells. Thus, it could be speculated that IL-6 overproduction in adiponectin-deficient mice might induce a favourable condition for γδ-T cells to differentiate and produce IL-17A in the development of skin inflammation. In fact, the past report investigating the function of adiponectin in the murine asthma model [50] also demonstrated a similar result to our data, demonstrating upregulated levels of IL-17A in association with IL-6 in lung tissues. Thus, hypoadiponectinemia, associated with IL-6 overproduction, could be responsible for IL-17A development and production. Chronic inflammation in adipose tissue accelerates obesity-related insulin resistance, leading to the development of the metabolic syndrome, including diabetes mellitus. Increasing evidence from human studies and animal experiments has established TNF-α as a main player of obesity-linked adipose inflammation [18] , [19] . Recently, besides the classic proinflammatory cytokine TNF-α, the role of IL-17 in adipose tissue and fat metabolism has been drawing attention [53] , [54] . Clinical studies have demonstrated that obese women exhibit increased levels of circulating IL-23 and IL-17, suggesting a potential role for IL-17 in obesity [55] . As comparable to human studies, several animal experiments indicate that obesity promotes Th17 expansion and subsequent IL-17 production, exacerbating disease severity in murine models of multiple sclerosis and inflammatory bowel disease, both of which are representative Th17-related diseases as well as psoriasis [56] . Furthermore, it has been reported that IL-17A production from PBMCs are increased in type 2 diabetes patients compared with healthy controls [57] , and percentage of haemoglobin A1c, a common clinical marker of diabetes severity, is positively correlated with IL-17 production [54] . Thus, IL-17 is now increasingly recognized as a new mediator of adipose tissue metabolism and inflammation, indicating that psoriasis and obesity-related metabolic disorders have a common immunopathological basis in disease development. Although the regulation of IL-17 by adiponectin was revealed by a murine model of psoriasiform dermatitis induced by imiquimod or IL-23, one of the problems in interpreting these data obtained from murine experiments is that chronicity are lacking and different cellular mediators from human psoriasis are involved in this model [34] . A murine model of imiquimod-induced psoriasiform dermatitis is indeed a powerful model to investigate the IL-17-related immunological pathway. However, this model describes an acute and simple skin inflammation, and thus, it has disadvantages in evaluating the maintenance of human chronic disease. Regarding cell types responsible for IL-17 production, γδ-T cells are main producers of IL-17 in a murine model of psoriasiform dermatitis [33] , [36] , whereas γδ-T cells take up a minority of IL-17-producing cells and conventional αβ-T cells produce most of IL-17 in the inflammation site of human psoriasis [58] , [59] . Thus, we also examined the effect of adiponectin on IL-17 production by human CD4- and CD8-positive T cells. In agreement with the results obtained from the murine experiments, IL-17 production by human CD4- or CD8-positive T cells was dose-dependently suppressed by adiponectin. Since adiponectin level was reduced at the skin, the actual site of inflammation, in psoriasis patients, decreased adiponectin would enhance IL-17 production from CD4- or CD8-positive T cells and finally exacerbate psoriasis dermatitis. Supplementation of adiponectin ameliorates disease progression induced by adiponectin deficiency in other several murine models [60] , [61] , [62] , suggesting that elevation of adiponectin level would be one of the strategies to improve the pathological condition of the disease. Consistent with past reports, exogenous adiponectin supplementation was effective to protect from dermatitis in adiponectin-deficient mice, but interestingly, it was not effective in wild-type mice. One possibility of this discrepancy in responsiveness between wild-type and adiponectin-deficient mice is that the effects of adiponectin might be elicited below a certain concentration and that, above that concentration, the effect might reach a plateau. Thus, it could be speculated that additional administration of exogenous adiponectin to wild-type mice might not have resulted in exerting biological effects. Adiponectin could be used as a potential therapeutic of dermatitis for those with low adiponectin levels, such as diabetic and obese patients, but not for those with sufficient adiponectin levels. In conclusion, adiponectin plays a crucial role to regulate psoriasis inflammation by directly suppressing IL-17 production from T cells. Our results provide a new therapeutic suggestion that increasing adiponectin levels after diet-induced weight loss would be efficient in improving psoriasis as well as metabolic disorders. Mice Original adiponectin-deficient mice (C57BL/6 and 129/Sv-mixed background) [63] were backcrossed with C57BL/6 mice more than seven times. Mice were 7–10 weeks old for all experiments. Age- and sex-matched wild-type C57BL/6 mice (CLEA Japan, Tokyo, Japan) were used as controls for adiponectin-deficient mice. All mice were maintained under a 12-h light/12 h dark cycle in a specific pathogen-free barrier facility. All studies and procedures were approved by the Committee on Animal Experimentation of Tokyo University. Induction of psoriasiform skin inflammation by imiquimod A daily topical dose of 62.5 mg of commercially available imiquimod cream (5%) (Beselna Cream; Mochida Pharmaceuticals, Tokyo, Japan) or control cream (Vaseline and a cream containing isostearic acid) was applied to the shaved back skin and ears of mice for 6 consecutive days (days 0–5). In some experiments, mice were intraperitoneally injected with mouse anti-IL-6 antibody (250 μg per mouse, R&D Systems, Minneapolis, MN), anti-IL-17 antibody (10 and 70 μg per mouse, R&D Systems) and control rat IgG (R&D Systems). The antibodies were injected 1 day before imiquimod application and day 1 (anti-IL-6 antibody) or day 2 (anti-IL-17 antibody). In the experiments of adiponectin supplementation, mice were given daily intraperitoneal injection of recombinant adiponectin (50 μg per day per mouse) [15] or PBS from 1 day before imiquimod treatment. Disease severity was assessed by using a scoring system based on the clinical Psoriasis Area and Severity Index, except for the affected skin area [32] . To be precise, erythema, scaling and thickening were scored independently on a scale from 0 to 4 (0, none; 1, slight; 2, moderate; 3, marked; 4, very marked), and the cumulative score was used as a total score (scale 0–12). Induction of psoriasiform skin inflammation by IL-23 Intradermal injections of 10 μl of PBS, either alone or containing 500 ng of recombinant mouse IL-23 (eBioscience, San Diego, CA) were performed into the dorsal aspect of the ear skin. Injections were performed every other day, and skin samples were collected 24 h after the second injection. Histological and immunohistochemical analyses Samples of naive or imiquimod-applied mouse back skin were collected. The samples were formalin-fixed and processed for standard haematoxylin and eosin staining. For immunohistochemistry, mouse skin was embedded in optimal cutting compound (OCT), snap-frozen in liquid nitrogen and stored at −80 °C. Cryosections were fixed with cold acetone for 5 min and incubated overnight at 4 °C with anti-mouse major histocompatibility complex class II antibody (1/50 dilution, Abcam, Cambridge, UK) or anti-mouse CD3 antibody (1/100 dilution, Abcam). Tissues were subsequently stained with an avidin–biotin peroxidase complex using a Vector ABC staining kit (Vector Laboratories, Burlingame, CA). Quantitative real-time reverse transcription–PCR analysis Total RNA was isolated from mouse back skin using RNeasy fibrous Tissue Mini kits (Qiagen, Germantown, MD) and complementary DNA was synthesized using Superscript III First strand synthesis kits (Invitrogen Life Technologies, Carlsbad, CA). Gene expression was quantified using the TaqMan gene expression assay (Applied Biosystems, Warrington, UK). Primers for TNF-α, IFN-γ, IL-6, IL-12p40, IL-23p19, IL-17A, IL-17F, IL-22 and glyceraldehyde 3-phosphate dehydrogenase (GAPDH) were available from Applied Biosystems. All samples were analysed in parallel for GAPDH gene expression as an internal control. The relative expression levels of each gene were determined by the 2 – ΔΔ CT method. PCR analysis for the Vγ chain Epidermal γδ-T cells and dermal γδ-T cells were sorted using FACS Aria II or III. Since a certain population of dermal γδ-T cells is recruited to the epidermis upon imiquimod treatment, epidermal γδ-T cells were collected before imiquimod treatment. Dermal γδ-T cells were collected after imiquimod application. Complementary DNA was synthesized and thermocycled for PCR amplification with 10 μM of each primer and 1.5 U of Taq polymerase (Invitrogen), using the following primers: Vγ4 5′-TGTCCTTGCAACCCCTACCC-3′, Vg5 5′-TGTGCACTGGTACCAACTGA-3′, Cγ 5′-CTTATGGAGATTTGTTTCAGC-3′, GAPDH 5'-AACTTTGGCATTGTGGAAGG-3′ and 5′-ACACATTGGGGGTAGGAACA-3'. The nomenclature of TCR Vγ chains is according to Garman [64] . Images have been cropped for presentation. Full-length gel images are shown in Supplementary Fig. 5 . Preparation of cells and flow cytometric analysis Skin samples applied with imiquimod or control cream for 5 days were incubated in 2 mg ml −1 Dispase (Gibco), and were separated into epidermis and dermis. Dermis was minced and then incubated with 2 mg ml −1 of collagenase type 2 (Worthington, Lakewood, NJ) in Tyrode buffer for 60–90 min. In some experiments, whole-skin samples were directly minced and digested mentioned above. The digested tissues were centrifuged, resuspended in PBS and filtered through a 70-μm mesh. Single-cell suspensions were stained on ice with either labelled monoclonal antibody or isotype control antibody. Cells were then analysed by FACSVerse flow cytometer (Becton Dickinson, San Jose, CA). The antibodies used were anti-CD3, γδTCR, Vγ4 and Vγ5 (1/100 dilution, Biolegend, San Diego, CA). In selected experiments, intracellular IL-17 staining was performed. Cells were stimulated with plate-bound anti-CD3e monoclonal antibody (BD Pharmingen, San Diego, CA) in the presence of PMA (Sigma, St Louis, MO), ionomycin and brefeldin A (1/1,000 dilution, Biolegend) for 4 h at 37 °C. Cells were first stained with each cell surface antibody and then fixed, permeabilized, followed by anti-mouse IL-17 monoclonal antibody staining (1/100 dilution, Biolegend). Thereafter, the cells were analysed. Cell sorting For analysis of in vitro experiments, dispase-separated epidermis and dermis were minced and digested as mentioned above, and the cells were sorted on a FACS Aria II or III with a purity of 97–99%. Immunoblotting Anti-AdipoR1 and AdipoR2 antibodies were obtained from Immuno-Biological Laboratories (Gunma, Japan). Sorted dermal γδ-T cells and human CD4- and CD8- T cells in lysis buffer were dissolved in NuPAGE LDS Sample Buffer with NuPAGE Sample Reducing Agent (Invitrogen) and denatured by heating for 5 min at 95 °C. Lysis buffer contained 20 mM Tris (pH 7.5), 150 mM NaCl, 1 mM EDTA, 1 mM EGTA, 1% Triton X-100, 2.5 mM sodium pyrophosphate, 1 mM glycerophosphate, 1 mM sodium orthovanadate, 1 mM phenylmethylsulphonyl fluoride and 1 μg ml −1 leupeptin. SDS–polyacrylamide gel electrophoresis was performed with NuPAGE 4–12% Bis-Tris gels and MES running buffer (Invitrogen). After transfer to an Immobilon-P transfer membrane (Millipore, Bedford, MA), the membrane was incubated for 1 h at room temperature with blocking buffer, overnight at 4 °C with the primary antibody, anti-AdipoR1 or AdipoR2 antibody (1/25 dilution), washed and incubated for 1 h at room temperature with the appropriate secondary antibody (1/2,000 dilution). After washing, visualization was performed by enhanced chemiluminescent techniques (Thermo Scientific, Rockford, IL). Images have been cropped for presentation. Full-length blotting images are shown in Supplementary Figs 6 and 7 . Secretion of IL-17 from dermal γδ-T cells Dermal γδ-T cells were sorted as mentioned above. Thereafter, γδ-T cells were cultured with complete medium (RPMI 1640 containing 10% FCS) overnight, and then were incubated with the indicated concentrations of adiponectin for 1 h, followed by treatment with IL-1β (10 ng ml −1 ; R&D systems) and IL-23 (5 ng ml −1 ; R&D systems) for another 24 h. The IL-17 protein levels in the supernatants were measured using an ELISA kit from R&D Systems according to the manufacturer’s direction. RNA interference for adiponectin receptors Accell siRNAs against AdipoR1 and AdipoR2, or nontargeting control siRNA were obtained from Thermo Fischer Scientific (Waltham, MA). All transfections were done using Accell siRNA Reagents following the manufacturer’s instructions (Thermo Fischer Scientific). Breifly, isolated γδ-T cells were incubated with Accell siRNA mixed with Accell siRNA delivery medium. After 72 h, transfected γδ-T cells were pretreated with adiponectin (10 μg ml −1 ) for 1 h, followed by treatment with IL-1β (10 ng ml −1 ) and IL-23 (5 ng ml −1 ) for another 6 h. Control experiments have revealed that AdipoR1 and AdipoR2 mRNA levels are reduced by >65%. Gene expression levels of IL-17A were quantified by real-time PCR as described above. Human subjects Subcutaneous adipose tissue and skin tissue samples were taken from both psoriasis patients and healthy controls. Samples were taken from 26 patients with psoriasis vulgaris (17 males and 9 females; aged: 51.8±11.9 years) before treatment and 12 healthy controls (8 males and 4 females; aged 49.8±9.4 years). All of the patients were diagnosed with clinical appearance and histological findings. Total RNA was then isolated using Trizol (Invitrogen), after which relative mRNA levels were determined using TaqMan gene expression assay as mentioned above. Institutional approval (University of Tokyo Graduate School of Medicine and Teikyo Universtiy School of Medicine) and written informed consent were obtained from all the subjects. Primers for human adiponectin and GAPDH were available from Applied Biosystems. Isolation and culture of PBMC PBMCs were obtained by density centrifugation over Ficoll-Paque (GE Healthcare, Buckinghamshire, UK) and were resuspended in RPMI 1640 supplemented with 10% fetal bovine serum. For IL-17 production, PBMCs were activated by plate-bound anti-CD3 (5 μg ml −1 ), soluble anti-CD28 (1 μg ml −1 ) and IL-23 (25 ng ml −1 ) by pretreatment with indicated concentrations of adiponectin for 1 h. For intracellular staining, PBMCs were incubated for 4 h with PMA and ionomycin in the presence of brefeldin A (all from Sigma) at 37 °C, and intracellular cytokine staining was carried out as mentioned above. The antibodies used were anti-CD4, CD8 and IL-17 (1/100 dilution, all from Biolegend). Statistical analyses Data obtained are presented as mean±s.e. Welch’s t -test was used for the statistical analysis of differences between two groups. One-way analysis of variance with Dunnett’s multiple comparison test was used for statistical analysis of the differences among multiple groups. Values of P <0.05 were considered to represent a significant difference. How to cite this article: Shibata, S. et al . Adiponectin regulates psoriasiform skin inflammation by suppressing IL-17 production from γδ-T cells. Nat. Commun. 6:7687 doi: 10.1038/ncomms8687 (2015).